Modulation-doped growth of mosaic graphene with single-crystalline p–n junctions for efficient photocurrent generation Device applications of graphene such as ultrafast transistors and photodetectors benefit from the combination of both high-quality p- and n-doped components prepared in a large-scale manner with spatial control and seamless connection. Here we develop a well-controlled chemical vapour deposition process for direct growth of mosaic graphene. Mosaic graphene is produced in large-area monolayers with spatially modulated, stable and uniform doping, and shows considerably high room temperature carrier mobility of ~5,000 cm 2 V −1 s −1 in intrinsic portion and ~2,500 cm 2 V −1 s −1 in nitrogen-doped portion. The unchanged crystalline registry during modulation doping indicates the single-crystalline nature of p–n junctions. Efficient hot carrier-assisted photocurrent was generated by laser excitation at the junction under ambient conditions. This study provides a facile avenue for large-scale synthesis of single-crystalline graphene p–n junctions, allowing for batch fabrication and integration of high-efficiency optoelectronic and electronic devices within the atomically thin film. Graphene, a single layer of hexagonal carbon framework with broadband photon absorption and extraordinary carrier mobility [1] , is attractive to high-performance electronic and optoelectronic devices, such as transistors [2] , [3] , [4] , [5] , optical modulators [6] and photodetectors [7] . Introduction of p–n junctions to graphene would allow for novel phenomena including Klein tunneling [8] , negative refractive index for Veselago lens [9] and even photoelectric conversion with a hot carrier-assisted photothermoelectric process [10] , [11] . However, existing methods for fabrication of graphene p–n junctions usually require external gate [10] or unstable adsorbed chemical dopants [12] , which are inconvenient for practical applications. In contrast, substitutional doping with heteroatoms via chemical vapour deposition (CVD) provides an effective route for simple and stable tuning of doping levels in graphene. Production of graphene via CVD growth on transition metal substrates has been steadily maturing [13] , [14] . Recently, N-doped graphene was successfully synthesized by mixing nitrogen compounds into forming gas during CVD growth [15] , [16] , [17] . Nevertheless, reported N-doped graphene typically has broad distribution of thicknesses, high-density of grain boundaries, and variations over dopant concentration and distribution. Moreover, selective-area substitutional doping of graphene is even more challenging, partly because traditional semiconductor selective doping techniques are less effective to this perfect atomically thin two-dimensional (2D) crystal formed by robust C–C bonds. It further hinders the creation of single-crystalline graphene p–n junction, which is of great significance for potential optoelectronic applications. Modulation doping, a technique to integrate of intricate n- and p-type segments in a tuned manner, is a powerful approach to achieve various nanostructure junctions with single-crystalline nature [18] . To improve the quality of N-doped graphene, we established a controlled growth technique to achieve modulation doping during the synthesis in single process. We have produced a novel mosaic graphene, a continuous graphene membrane with uniform thickness and regionally varied doping profile. Growth of modulation-doped mosaic graphene The schematic structure as well as its growth procedure of modulation-doped mosaic graphene is shown in Fig. 1a . To initiate the growth, discrete intrinsic graphene grains with typical diameter of ~10 μm were first grown on an annealed polycrystalline copper substrate at 1,000 °C [13] ( Supplementary Fig. S1 ). These discrete grains would serve as matrices for the following grafting stage. After a short purging period, acetonitrile vapour was introduced as precursor gas for the laterally grafted growth of N-doped graphene [15] ( Supplementary Fig. S2 ). As the space between the intrinsic grains was previously controlled, spontaneous nucleation of N-doped graphene grains is successfully suppressed ( Supplementary Fig. S3 ). Coalescence of grains eventually yields a continuous monolayer mosaic graphene film with uniform contrast under optical microscope (OM) ( Fig. 1b ). As shown in the scanning electron microscope (SEM) image ( Fig. 1c ), bright polygonal islands corresponding to intrinsic graphene grains were clearly recognized, surrounded by dark intervals with substitutionally doped nitrogen atoms. The sample is predominantly of monolayer coverage due to the suppression of graphene adlayers on copper [13] . In addition, once seeds for intrinsic grains were specifically predefined [19] , the consequent growth of mosaic grains can be as well templated, thus leading to the creation of periodic mosaic graphene superlattice structure ( Fig. 1d and Supplementary Fig. S4 ). 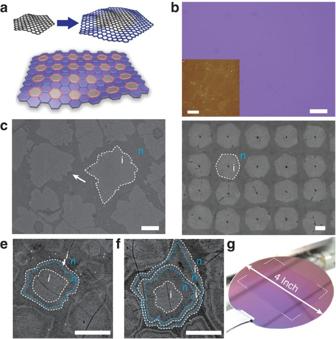Figure 1: Synthesis and morphology of modulation-doped graphene. (a) Top: schematic drawing of modulation doping growth. The nucleation and expanding stages were grown with alternate forming gases. Bottom: schematic diagram of mosaic graphene, where pixels with different colours represent graphene with different doping levels. (b) OM image of mosaic graphene transferred onto 300 nm SiO2/Si substrate. Scale bar, 10 μm. Inset: AFM image of mosaic graphene. Scale bar, 5 μm. (c,d) Typical SEM images of random and ordered mosaic graphene, respectively. Intrinsic and N-doped portions can be identified by the contrast. Scale bars, 2 μm. (e,f) Typical SEM images with two and three modulation cycles, respectively. These high-order structures behave as irregular homocentric disks with radial doping modulations. Scale bars, 2 μm. (g) Large-area mosaic graphene transferred onto a 4-inch silicon wafer. Figure 1: Synthesis and morphology of modulation-doped graphene. ( a ) Top: schematic drawing of modulation doping growth. The nucleation and expanding stages were grown with alternate forming gases. Bottom: schematic diagram of mosaic graphene, where pixels with different colours represent graphene with different doping levels. ( b ) OM image of mosaic graphene transferred onto 300 nm SiO 2 /Si substrate. Scale bar, 10 μm. Inset: AFM image of mosaic graphene. Scale bar, 5 μm. ( c , d ) Typical SEM images of random and ordered mosaic graphene, respectively. Intrinsic and N-doped portions can be identified by the contrast. Scale bars, 2 μm. ( e , f ) Typical SEM images with two and three modulation cycles, respectively. These high-order structures behave as irregular homocentric disks with radial doping modulations. Scale bars, 2 μm. ( g ) Large-area mosaic graphene transferred onto a 4-inch silicon wafer. Full size image More complex mosaic graphene structures were achieved through multiple modulation cycles with period tuning. Figure 1e shows typical SEM images of the mosaic graphene with two and three modulation cycles, respectively. Spatially well-defined intrinsic and N-doped portions are clearly recognized as homocentric growth rings with alternating contrast. The observation of sharp junction interface indicated the lateral extension growth and the high thermal stability of N-doped portion. The width of either well-defined portion can be as narrow as several hundred nanometres. On the other hand, wafer-sized monolayer mosaic graphene was successfully synthesized ( Fig. 1g ), which can be further scaled up for batch production of mosaic graphene, by using larger vessel and copper foil, or the roll-to-roll process [14] . Spectroscopic characterizations of modulation-doped mosaic graphene The concentration and uniformity of doping in either side of the lateral junctions, as well as the width of depletion region, are important for the performance of p–n junction. To explore this, mosaic graphene grown on copper substrate was characterized by both photoemission electron microscope (PEEM) and low-energy electron microscope (LEEM) under ultrahigh vacuum. As the photoemission threshold strongly depends on the position of Fermi level, doping modulation would lead to variations in the productivity of photoelectrons [20] . As a result, the intrinsic graphene portion with higher work function exhibited relatively darker image contrast compared with N-doped portion in the PEEM image ( Fig. 2a ). A clear boundary at the lateral junction of mosaic graphene was observed in the PEEM image. The profile line in Fig. 2a reveals the variation of work function across graphene lateral junction. Despite the fluctuations in both portions, the profile exhibited an abrupt rise within 80 nm at the junction interface, indicating the sharpness of the lateral junction. Similar with SEM, intrinsic portions in the same area of the mosaic graphene sample exhibited relatively lighter contrast in LEEM image taken at start voltage of 1.70 V ( Fig. 2b , inset). While the energy of incident electron is increasing from 0 eV, the reflected intensity I gradually drops from I 0 . The threshold electron energy at which relative reflectivity I / I 0 decreases to 0.9 can be used to identify the work function of graphene [21] , [22] . We accordingly found the work function of intrinsic and N-doped graphene within the same copper grain differed for ~0.2 eV at 330 K ( Fig. 2b ). 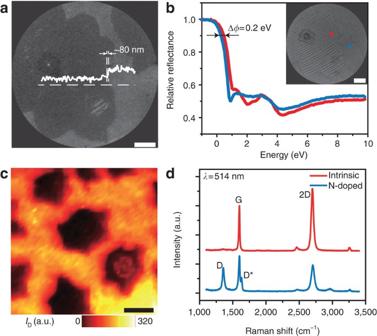Figure 2: Spectroscopy characterizations of modulation-doped graphene. (a) PEEM image of mosaic graphene on Cu foil with start voltage of 0.0 V. Intrinsic graphene with higher work function exhibited darker contrast. The line profile of contrast is collected along the dashed line. Scale bar, 2 μm. (b) Relative electron reflectivity data recorded at the identified spots of mosaic graphene shown in the inset. The derivation between the two curves corresponds to their difference in work function. Inset: LEEM image of mosaic graphene with start voltage of 1.70 V. Scale bar, 2 μm. (c) D band mapping of Raman spectroscopy over a certain region of mosaic graphene transferred on a SiO2substrate, revealing the distribution of two portions. Scale bar, 5 μm. (d) Typical Raman spectra of intrinsic and N-doped portions of mosaic graphene collected with 514 nm incident laser. Figure 2: Spectroscopy characterizations of modulation-doped graphene. ( a ) PEEM image of mosaic graphene on Cu foil with start voltage of 0.0 V. Intrinsic graphene with higher work function exhibited darker contrast. The line profile of contrast is collected along the dashed line. Scale bar, 2 μm. ( b ) Relative electron reflectivity data recorded at the identified spots of mosaic graphene shown in the inset. The derivation between the two curves corresponds to their difference in work function. Inset: LEEM image of mosaic graphene with start voltage of 1.70 V. Scale bar, 2 μm. ( c ) D band mapping of Raman spectroscopy over a certain region of mosaic graphene transferred on a SiO 2 substrate, revealing the distribution of two portions. Scale bar, 5 μm. ( d ) Typical Raman spectra of intrinsic and N-doped portions of mosaic graphene collected with 514 nm incident laser. Full size image To determine the quality and the spatial distribution of dopant in mosaic graphene, we conducted Raman mapping of mosaic graphene transferred on a SiO 2 /Si substrate. As illustrated in Fig. 2c , the D band intensity map revealed a polygonal pattern with dark cores surrounded by bright loops. The uniformity of doping was again confirmed through the distribution of D band intensity. Full spectra of both portions were collected and illustrated in Fig. 2d . The spectrum exhibited sharp G and 2D Raman bands with a ratio I G / I 2D <1 was recognized as intrinsic graphene [23] . The absence of the D band indicates that the high quality of intrinsic graphene was preserved despite of the following N-doped growth. In contrast, the region exhibited strong D and D* bands, as well as broadening and shifting of both G band and 2D band in its spectrum ( Supplementary Fig. S5 ) can be ascribed to N-doped portion [24] , [25] . Structural characterizations of modulation-doped mosaic graphene The quality of graphene junction between intrinsic and N-doped portions is crucial for carrier conduction as well as efficient photocurrent generation and collection. Especially, single-crystalline junction would provide much better performance with less carrier scattering than grain boundaries in polycrystalline graphene [19] . To this end, we prepared discrete mosaic graphene grains, by halting the growth before full coverage in the stage of N-doped graphene, which facilitates investigation of the interfacial structure after locating the lateral junction. From the SEM image ( Fig. 3a ), we confirmed that these discrete grains consist of intrinsic cores and ~2 μm wide N-doped edges. The specific shape as well as the width of the edge could serve as marks for the locating of the lateral junction with atomic force microscopy (AFM) and transmission electron microscopy (TEM). Consistent with the OM image, the interface identified by the dashed line showed ideal smoothness in AFM ( Fig. 3b and Supplementary Fig. S6 ), with no observable crack or overlap. To further confirm the single-crystalline essence of the junction, samples from the same batch were characterized by TEM and selected area electron diffraction (SAED). Ultra-thin (~5 nm thick) porous carbon membrane was used to support these discrete grains. In Fig. 3c , graphene grains were identified through the slight contrast from the support. Along the white dashed arrow in Fig. 3c , extensive SAED patterns were captured with ~600 nm aperture and incident beam normal to the sample. Six typical SAED patterns among them were illustrated ( Fig. 3d ), taken from the positions labelled in Fig. 3c , which together confirmed the single-crystalline nature of the discrete grain. The first and the last patterns were collected within ~2 μm from the edge correspond to the N-doped portion, whereas the other four lie in the intrinsic portion. It is worth noting that these patterns exhibit the same orientations of ~10° as labelled in Fig. 3d . The thickness of the sample was further confirmed to be monolayer by analysing line profile of the diffraction pattern in Fig. 3d [26] . Histogram of pattern orientation distributions from extensive SAED studies shown in Fig. 3e exhibited two pronouncing peaks separated by <1°, which could be reasonably ascribed to the wrinkle in the centre of the grain ( Fig. 3c ). Moreover, lattice distance of the sample could also be obtained from SAED patterns. The histogram in Fig. 3f reveals an average lattice distance of ~2.43 Å. These structural observations conclude that the crystal registry is retained during modulation doping growth of mosaic graphene, yielding single-crystalline lateral p–n junctions. 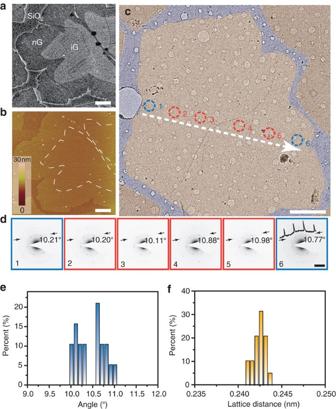Figure 3: Structural studies of modulation-doped graphene. (a) SEM image of a discrete modulation-doped graphene grain. Scale bar, 2 μm. (b) AFM image of the specific area ina. The dashed line outlines intrinsic portion of the grain. Scale bar, 2 μm. (c) Low-magnification TEM image of a discrete mosaic graphene grain. Graphene grains and supporting membrane are rendered orange and purple, respectively. The white dashed arrow indicated the direction along which SAEDs were performed. The six circles presented positions where SAED patterns indwere collected. Observed pores belong to the supporting membrane rather than graphene sample. Scale bar, 2 μm. (d) SAED patterns of specified spots inc. The number labelled the angle along the arrow pair in each panel. In the last panel, intensity section along the diffraction pattern was plotted. Scale bar, 5 nm−1. (e) Histogram of angle distribution from extensive SAED patterns within the grain. (f) Histogram of lattice distance distribution obtained from SAED patterns within the grain. Figure 3: Structural studies of modulation-doped graphene. ( a ) SEM image of a discrete modulation-doped graphene grain. Scale bar, 2 μm. ( b ) AFM image of the specific area in a . The dashed line outlines intrinsic portion of the grain. Scale bar, 2 μm. ( c ) Low-magnification TEM image of a discrete mosaic graphene grain. Graphene grains and supporting membrane are rendered orange and purple, respectively. The white dashed arrow indicated the direction along which SAEDs were performed. The six circles presented positions where SAED patterns in d were collected. Observed pores belong to the supporting membrane rather than graphene sample. Scale bar, 2 μm. ( d ) SAED patterns of specified spots in c . The number labelled the angle along the arrow pair in each panel. In the last panel, intensity section along the diffraction pattern was plotted. Scale bar, 5 nm −1 . ( e ) Histogram of angle distribution from extensive SAED patterns within the grain. ( f ) Histogram of lattice distance distribution obtained from SAED patterns within the grain. Full size image Transport properties of modulation-doped mosaic graphene Fundamental transport measurements were performed to evaluate the electronic properties of our modulation-doped graphene, in particular to verify the single-crystalline lateral junction. Continuous mosaic graphene film transferred onto a silicon substrate with SiO 2 as back gate was etched into narrow strips, and then embedded with four-probe configuration ( Fig. 4a , inset). Resistance of both portions and the junction are measured at room temperature. As shown in Fig. 4a , N-doped portion exhibited larger resistance than intrinsic, arising from scattering defects. However, resistance across lateral junction is quite similar with that of intrinsic portion. The absence of scattering at the junction evidently indicates the high quality of the lateral junction, resulting from the single-crystalline essence. Moreover, graphene p–n junction exhibited no rectification effect as expected because of the absence of effective band gap, as indicated by the output properties shown in Supplementary Fig. S7 . Transfer properties of mosaic graphene are further studied as shown in Fig. 4b and Supplementary Fig. S8 . Gate sweeping of each portion produced a single peak in resistivity. The distance between two charge neutrality points (Dirac points) corresponds to an electron doping concentration of n d ~2.70 × 10 12 cm −2 . This result resonates well with the work function difference measured by LEEM through the relation (ref. 27 ). Transfer characteristic across the interface exhibits two separated peaks, hallmark of a graphene p–n junction. We further extracted carrier mobility near each Dirac point from these curves. Surprisingly, the room temperature mobility of the N-doped portion can be as high as 2,500 (holes) and 1,800 (electrons) cm 2 V −1 s −1 , comparable to that of the intrinsic portion (4,000 cm 2 V −1 s −1 for holes and 2,500 cm 2 V −1 s −1 electrons). Extensive study on other 10 devices yielded a mobility of 1,000–2,500 cm 2 V −1 s −1 for N-doped and 2,500–5,000 cm 2 V −1 s −1 for intrinsic graphene, respectively. Such mobility of N-doped graphene is over 1–2 orders of magnitude higher than that in previous reports [16] . In conventional CVD growth of N-doped graphene, the density of spontaneous nucleation is remarkably high ( Supplementary Fig. S9 ), yielding massive scattering grain boundaries. In contrast, grain boundaries in our N-doped mosaic graphene are limited by predefined intrinsic grains, yielding high-carrier mobility with less grain boundary scattering [28] . 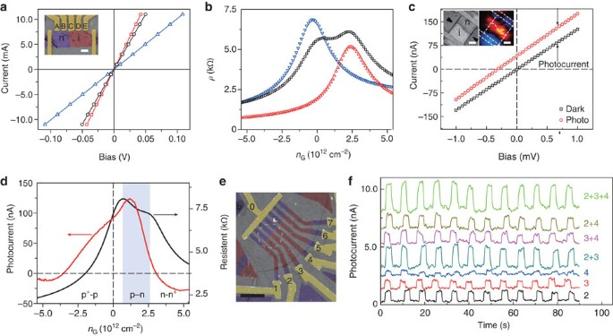Figure 4: Transport and photoelectric properties of mosaic graphene. (a) Representative I–V curves at room temperature measured within either component and cross the p–n junction. Inset: SEM image of measured device, with intrinsic and N-doped graphene false coloured into red and blue, respectively. Scale bar, 2 μm. (b) Transfer properties of the same device measured with four-probe configuration. Both intrinsic (red up-triangle) and N-doped (blue down-triangle) portions exhibited separated single Dirac point, whereas the p–n junction (black square) produced a representative curve with two Dirac points. (c) Current versus source-drain bias with (red square) and without (black square) 633 nm laser beam focused at the p–n junction. The difference between the two curves represents the photocurrent. Inset: SEM image of the device (left) and corresponding photocurrent mapping image (right) collected with +15 V gate bias, with electrodes and graphene channel indicated as dashed lines. Scale bars, 2 μm. (d) Transfer (black) and photoelectric (red) measurements of p–n junction in mosaic graphene. (e) False coloured SEM image of graphene photodetector array. Individual channels were labelled from 1 to 7, sharing the same source and controlled by corresponding switches. The dashed circle represents the size and position of laser spot. Scale bar, 5 μm. (f) Photoresponses of individual channels and their additions are shown as different curves. Figure 4: Transport and photoelectric properties of mosaic graphene. ( a ) Representative I–V curves at room temperature measured within either component and cross the p–n junction. Inset: SEM image of measured device, with intrinsic and N-doped graphene false coloured into red and blue, respectively. Scale bar, 2 μm. ( b ) Transfer properties of the same device measured with four-probe configuration. Both intrinsic (red up-triangle) and N-doped (blue down-triangle) portions exhibited separated single Dirac point, whereas the p–n junction (black square) produced a representative curve with two Dirac points. ( c ) Current versus source-drain bias with (red square) and without (black square) 633 nm laser beam focused at the p–n junction. The difference between the two curves represents the photocurrent. Inset: SEM image of the device (left) and corresponding photocurrent mapping image (right) collected with +15 V gate bias, with electrodes and graphene channel indicated as dashed lines. Scale bars, 2 μm. ( d ) Transfer (black) and photoelectric (red) measurements of p–n junction in mosaic graphene. ( e ) False coloured SEM image of graphene photodetector array. Individual channels were labelled from 1 to 7, sharing the same source and controlled by corresponding switches. The dashed circle represents the size and position of laser spot. Scale bar, 5 μm. ( f ) Photoresponses of individual channels and their additions are shown as different curves. Full size image Photocurrent generation at graphene p–n junction The remarkably high mobility of our mosaic graphene with high-quality p–n junctions facilitates the generation of efficient photocurrent under illumination. As a demonstration, one grain of modulation-doped graphene was patterned and embedded into a two-terminal device ( Fig. 4c , inset). A focused 632.8nm laser spot (~1 μm, ~900 μW) was used to excite photocarriers. As illustrated in Fig. 4c , the p–n junction produced a pronounced current shift when illuminated by laser, indicating its capability of photoelectric conversion. We further conducted photocurrent mapping of the device ( Fig. 4c , inset). It was clearly observed that photocurrent was generated over the junction, as well as the two electrodes, with contrary directions. Moreover, the intensity of photocurrent generated at the junction is approximately two times stronger than that at the graphene/electrodes junctions, indicating higher efficiency for potential photodetector applications. The photocurrent of p–n junction as function of carrier concentration was plotted together with the resistance in Fig. 4d . The resistance followed a typical curve with two neutral points, separating the whole curve into three regimes labelled n-n + , p–n and p + -p. Meanwhile, the photocurrent curve exhibited a single peak with two polarity reversals, in contrast to those at source and drain electrodes, both of which reversed only once as indicated in Supplementary Fig. S10 . Moreover, the region whose photocurrent is determined by p–n junction could span over 2 μm along the channel. The maximum current of ~125 nA pinned between the two neutral points in the p–n regime, when laser is right positioned at the junction. The polarity reversal of the photocurrent is in contradiction with traditional photovoltaic process in which excited carriers were separated solely by the built-in electric filed, as the polarity of p–n junction remained unchanged during tuning of the global gate voltage. To understand the reversal, photothermoelectric effect [10] is considered as the primary scheme, where hot carriers excited by photon eventually result in thermoelectricity. The photovoltage is determined by the temperature difference Δ T of electrons inside and outside the excited zone. Considering the Seebeck coefficient of graphene (~100 μV K −1 ) at room temperature [29] , Δ T was estimated to be approaching 10 K in our case. The efficiency of photocurrent generation relies on the photon absorption and excitation rate of carriers, as well as the separation of excitons. In our case, the unbiased photocurrent responsivity of ~0.1 mA W −1 is mainly impeded by the large channel resistance as well as energy dissipation through the substrate. On the other hand, carrier multiplication predicted theoretically [30] may further improve the carrier excitation rate in graphene. Enhancement of absorption through plasmonic resonance [31] , [32] or microcavity [33] could also help to increase the absolute response of monolayer graphene. We further studied integration of multiple graphene photodetector channels, as a model device for multiple signal computing. A photodetector array with seven individual p–n junction channels was fabricated monolithically from a single graphene hybrid domain ( Fig. 4e ). A laser spot with ~5 μm in diameter shone over three p–n junction channels to produce photocarriers. Depending on the status of corresponding peripheral switches, cooperative photodetection was achieved. Signals from individual channels as well as their additions were shown in Fig. 4f . It thus confirmed the reliability as well as stability of these photodetectors based on single-crystalline graphene p–n junctions. In addition, the photocurrent strength generated by each individual channel is proportional to the power of illuminating light, suggesting the possibility of imaging with spatial resolution. In summary, we have established a modulation doping technique for controlled growth of mosaic graphene with spatially well-defined dopant and single-crystalline p–n junctions. The sample showed excellent transport properties in both intrinsic and N-doped portions. High-quality p–n junctions between two portions can be used for efficient photocurrent generation under the photothermoelectric scheme. Arising from the improved doping, mosaic graphene would benefit not only graphene based photocurrent generation but also fuel cells [34] , lithium batteries [15] and even supercapacitors [35] . Mosaic graphene growth and transfer Large-area mosaic graphene was grown on annealed copper foil loaded inside a homemade low-pressure CVD system, with methane and acetonitrile vapour for intrinsic and N-doped portions, respectively. The sample was then transferred to silicon wafer covered with silicon oxide with the aid of poly(methyl methacrylate). Detailed growth procedure could be found in Supplementary Methods . Characterizations of mosaic graphene Characterizations were done with OM (Olympus BX51), SEM (Hitachi S-4800, acceleration voltage 5–30 kV), AFM (DI Nanoscope IIIa), Raman spectrum (Horiba, LabRAM HR-800) and TEM (FEI Tecnai T20, acceleration voltage 200 kV). PEEM and LEEM were carried out in an Elmitec LEEM/PEEM system with an aberration corrector under ultrahigh vacuum of ~1 × 10 −10 Torr. The PEEM image was acquired with a mercury lamb. Device fabrication Mosaic graphene was first transferred onto a silicon substrate with silicon oxide as dielectric layer. SEM was used to identify specific regions, while p–n junction from the same domain is preferred. Standard EBL (STRATA DB235, FEI) was carried out to define micro patterns. Designed graphene strips were shaped by plasma etching. Afterward, trilayer metal electrodes (0.5 nm Cr/25 nm Pd/10 nm Au) were deposited by thermo/e-beam/thermo evaporation (UNIVEX 300, Leybold Vacuum) in one batch. The device was lifted-off by acetone and washed with isopropanol. Finally, it was blow dried with nitrogen gas. Transport measurement A homemade spherical chamber combined with turbo station (Pfeiffer, HiCube 80 Eco) provided high-vacuum environment for the transport measurement of graphene p–n junction. Overnight pumping was usually required to achieve the intrinsic performance. Baking was carefully avoided in case of any potential damage. A semiconductor analyser (Keithley, SCS-4200) was used to measure the four terminal electrical properties with Keithley 6517A providing gate bias. Photocurrent measurement Photocurrent from graphene p–n junction was measured on a modified Raman spectrometer (Renishaw-1000). Electrical cables were equipped to extract photocurrent to the semiconductor analyser (Keithley, SCS-4200). A 632.8-nm Griot He–Ne laser was focused through an Olympus BH2 OM. Microstage on the Raman spectrometer is used for alignment with accuracy better than 0.1 μm. How to cite this article: Yan, K. et al. Modulation-doped growth of mosaic graphene with single-crystalline p–n junctions for efficient photocurrent generation. Nat. Commun. 3:1280 doi: 10.1038/ncomms2286 (2012).